Identifying the nature of the active sites in methanol synthesis over Cu/ZnO/Al2O3catalysts 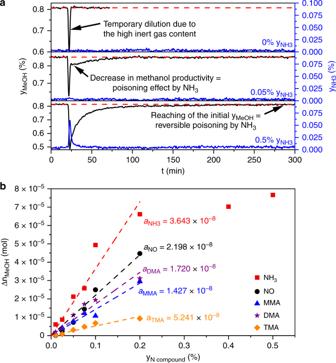Fig. 1: High-pressure pulse experiments and the determined inhibition strengths. aRecorded methanol (black curves) and NH3(blue curves) mole fractions during the injection of pulses with different NH3partial pressures over the Cu/ZnO/Al2O3catalyst (conditions: 210 °C, 60 bar, 13.5% CO, 3.5% CO2, 73.5% H2, 9.5% N2).bCorrelation of the determined ΔnMeOH(non-produced amount of methanol over a defined period of time) values (Supplementary Note1) with the injected mole fractions of the investigated N compounds (NH3red squares and line, NO black points and line, monomethylamine (MMA) blue triangles and line, dimethylamine (DMA) violet stars and line, trimethylamine (TMA) orange diamonds and line). The corresponding pulse experiments are shown in Supplementary Figs.1–5.a, the slope of the corresponding linear interpolation, is defined as the inhibition strength. The heterogeneously catalysed reaction of hydrogen with carbon monoxide and carbon dioxide (syngas) to methanol is nearly 100 years old, and the standard methanol catalyst Cu/ZnO/Al 2 O 3 has been applied for more than 50 years. Still, the nature of the Zn species on the metallic Cu 0 particles (interface sites) is heavily debated. Here, we show that these Zn species are not metallic, but have a positively charged nature under industrial methanol synthesis conditions. Our kinetic results are based on a self-built high-pressure pulse unit, which allows us to inject selective reversible poisons into the syngas feed passing through a fixed-bed reactor containing an industrial Cu/ZnO/Al 2 O 3 catalyst under high-pressure conditions. This method allows us to perform surface-sensitive operando investigations as a function of the reaction conditions, demonstrating that the rate of methanol formation is only decreased in CO 2 -containing syngas mixtures when pulsing NH 3 or methylamines as basic probe molecules. The high consumption of fossil fuels causes the emission of greenhouse gases and enhances global warming. Therefore, it is the aim of current research to find alternative energy sources and renewable raw materials. One possible alternative is methanol, which is used in a wide range of applications as basic chemical, fuel additive as well as energy carrier [1] , [2] . It has a high potential to substitute hydrocarbons originating from fossil fuels in many areas [3] . Nowadays, methanol is still industrially produced by the heterogeneously catalysed conversion of syngas, a gas mixture containing CO, CO 2 and H 2 obtained from natural gas or coal, over Cu/ZnO/Al 2 O 3 catalysts at elevated temperatures and pressures [4] . For a methanol production with low CO 2 footprint, the mixing of exhaust gases from steel production with sustainably produced H 2 from water electrolysis is a promising route to achieve the gas composition of conventional syngas mixtures [5] . However, many known and unknown impurities in the ppm as well as in the ppb range may be present in such an off-gas-derived syngas, and the effects of most impurities on the catalytic activity, selectivity and stability cannot be predicted with certainty in view of the lack of poisoning studies in literature [6] , [7] . These impurities can interact as irreversible poisons, which strongly interact with the active sites, or as reversible poisons, which can be desorbed from the active sites and flushed out of the reactor [8] , [9] . In case of reversible poisoning, the poisons can act as selective probe molecules adsorbing on the active sites without irreversible deactivation. Thus, selective poisoning may allow gaining new insight in the nature of the active sites [10] . The active site for methanol formation of the industrial Cu/ZnO/Al 2 O 3 catalyst has been under debate over the last decades. Recent models are the Cu 0 –Zn 0 surface alloy proposed by the Nakamura and Chorkendorff groups [11] , [12] , Zn δ+ species at the defective Cu 0 surface claimed by the Schlögl group [13] , graphitic-like ZnO x layer on the Cu 0 particles also suggested by the Schlögl group [14] , and ZnO on the top layer of the Cu 0 particles postulated by the Rodriguez group [15] . All models are based on strong metal support interactions (SMSI) [16] resulting in Cu–Zn interface sites that are essential for a highly active catalyst, but they differ in the nature of the Zn species in close contact with Cu 0 , which are controversially debated to be metallic or positively charged. The most active site of methanol synthesis is described as metallic Zn species alloyed into defined Cu 0 steps [13] . Furthermore, it is proposed that high coverages of oxygen-containing intermediates like formate only exist under industrially relevant high-pressure conditions and lead to a partial oxidation of the metallic Zn sites due to the oxophilic nature of Zn compared with Cu 0 [13] . However, there is no characterisation method available for the Cu/ZnO/Al 2 O 3 catalyst typically operated above 200 °C and 50 bar [4] , which is able to identify this oxidising effect, because the adjustment of both high-temperature and high-pressure conditions and surface sensitivity is technically impossible for typical single-crystal investigations [11] , transient in situ experiments [17] , [18] , adsorption and desorption studies [12] , [19] , in situ infrared (IR) spectroscopy [11] , [20] , N 2 O frontal chromatography [12] , [19] , X-ray photoelectron spectroscopy (XPS) [11] , [12] , [15] , [19] , ambient pressure XPS [13] , neutron scattering [13] , microcalorimetry [21] , [22] , scanning tunnelling microscopy [11] , in situ IR reflection-absorption spectroscopy [11] , high-resolution transmission electron microscopy (TEM) [14] , [23] , in situ TEM [24] , electron energy loss spectroscopy [14] , in situ X-ray absorption spectroscopy [16] , or operando X-ray diffraction [25] . To confirm the positive charge of the Zn species in close contact with Cu 0 , we establish a surface-sensitive operando method, which allows us to inject selective reversible poisons as probe molecules such as NH 3 into the syngas feed. By applying this high-pressure pulse unit (HPPU), we are able to identify the nature of the active sites of the working Cu/ZnO/Al 2 O 3 catalyst under industrially relevant conditions. In detail, we perform conventional methanol synthesis over an industrial Cu/ZnO/Al 2 O 3 catalyst with CO/CO 2 -containing syngas mixtures above 200 °C and at 60 bar. We investigate the reversible poisoning mechanism of NH 3 as well as of different types of methylamines and define the corresponding inhibition strength by the non-produced amount of methanol over a defined period of time. Parallel to the reversible poisoning by the amines, we co-feed ethylene into the syngas mixture, which is fast hydrogenated to ethane, we investigate the reversible poisoning mechanism of NO, and we change the syngas mixture from CO 2 - to CO-free gas mixtures to clearly confirm that the methanol synthesis catalyst exposes both highly active Cu 0 –Zn δ+ sites and metallic Cu 0 sites. At the end, the obtained results are discussed in view of the controversial debate on the active site in methanol synthesis demonstrating that the chosen reaction conditions and the time on stream (TOS) control the structure of the catalyst surface. High-pressure pulse experiment (HPPE) The self-built HPPU enabled us to inject defined amounts of probe molecules as pulses into the syngas stream under methanol synthesis conditions (210 °C, 60 bar). In this way, a variety of valuable kinetic results can be collected in a short period of time without disturbing the main reaction on the surface sites for a too long period of time to minimize possible irreversible structural transformations. When injecting N-containing compounds acting as reversible poisons, the temporary blocking of active sites only occurs when the poison is present in the feed gas stream, which is exemplarily shown for NH 3 in Fig. 1a . Fig. 1: High-pressure pulse experiments and the determined inhibition strengths. a Recorded methanol (black curves) and NH 3 (blue curves) mole fractions during the injection of pulses with different NH 3 partial pressures over the Cu/ZnO/Al 2 O 3 catalyst (conditions: 210 °C, 60 bar, 13.5% CO, 3.5% CO 2 , 73.5% H 2 , 9.5% N 2 ). b Correlation of the determined Δn MeOH (non-produced amount of methanol over a defined period of time) values (Supplementary Note 1 ) with the injected mole fractions of the investigated N compounds (NH 3 red squares and line, NO black points and line, monomethylamine (MMA) blue triangles and line, dimethylamine (DMA) violet stars and line, trimethylamine (TMA) orange diamonds and line). The corresponding pulse experiments are shown in Supplementary Figs. 1 – 5 . a , the slope of the corresponding linear interpolation, is defined as the inhibition strength. Full size image A typical HPPE consists of three steps: First, steady state with clean syngas has to be established. The second step is the injection of the probe molecule as a pulse passing through the catalyst bed, and in the third step the period of time is determined until the initial rate of methanol formation is recovered. The pulsing of pure N 2 (0% NH 3 in Fig. 1a ) illustrates that the used low mole fractions of reversible poisons as well as the high inert content in the sample loop lead to a temporary dilution of the product stream. This sharp negative pulse present in every HPPE is neglected for the interpretation of the results. The rising partial pressure of NH 3 leads to an increasing loss of methanol activity after the temporary dilution and to longer regeneration times. In addition to the methanol mole fraction (black curves), the NH 3 mole fractions (blue curves) were also monitored. For the experiment with 0.05% NH 3 , no NH 3 signal was detected, since it is converted to the methylamines monomethylamine (MMA), dimethylamine (DMA) and trimethylamine (TMA) (Supplementary Fig. 10 ) reacting with oxygen-containing intermediates of methanol synthesis such as formate [26] , [27] . This means that the NH 3 signal of the 0.5% HPPE represents the part of the injected NH 3 , which does not interact with the catalyst surface, because the position of the signal is equal to the temporary dilution. Obviously, the adsorbed NH 3 species and syngas reactants are part of adsorption equilibria, so that a complete deactivation of methanol synthesis is not possible with a reversible poison in contrast to an irreversible one [8] , [28] . In the same way, MMA (Supplementary Fig. 2 ), DMA (Supplementary Fig. 3 ) as well as TMA (Supplementary Fig. 4 ) were also injected as pulses into the feed gas stream under high-pressure conditions to better understand the reversible poisoning mechanism of NH 3 . NO was also used (Supplementary Fig. 5 ), which is hydrogenated to NH 3 and H 2 O (Supplementary Fig. 11 ). All investigated N compounds act as reversible poisons, and for the comparison of the different poisoning strengths the relevant methanol mole fractions were integrated to obtain the non-produced amount of methanol Δ n MeOH during the required period of regeneration time (Supplementary Note 1 , Supplementary Fig. 6 ). The correlation of the calculated values Δ n MeOH with the different mole fractions of the reversible poisons is shown in Fig. 1b . The Δ n MeOH values for every corresponding poison correlate linearly with the mole fraction of the poison for values below 0.2% under the investigated conditions. Above this mole fraction, the poisoning strength reaches a stationary regime due to the limited deactivation effect of reversible poisons, exemplarily shown for NH 3 (injection of 0.4 and 0.5%). The linear trend of the curves in Fig. 1b can be easily predicted with a one-parameter function through the origin. Here, the slope is defined as the inhibition strength a , and the corresponding values are shown in Fig. 1b . When comparing the determined values for the individual inhibition strengths, the following sequence is obtained, in which NH 3 is the strongest reversible poison and TMA the weakest: 
    NH_3 > NO > DMA≈MMA > TMA. (1) The consecutive reaction of NH 3 to TMA is one reason for this correlation. NH 3 requires the highest number of methylation steps until the final product TMA is formed, resulting in the longest blocking of active sites as well as in the highest consumption of oxygen-containing intermediates [26] , [27] . In contrast, TMA only blocks the active sites by adsorption, since no further methylation is possible (Supplementary Fig. 10b ), leading to the shortest residence time on the surface and the lowest inhibition strength. In principle, MMA should be a stronger poison than DMA, but Fig. 1b shows that the inhibition strength of DMA is only slightly higher. Thus, it can be assumed that the methylation steps are fast and a clear distinction between both methylamines is difficult to identify at 210 °C and not observable at 250 °C (Supplementary Fig. 10b ). The inhibition strength of NO should also be higher than that of NH 3 due to the additional hydrogenation step, but the poisoning by NH 3 and NO proceeds in different ways as explained in Fig. 2 . Fig. 2: Continuous dosing experiments coupled with HPPEs. a Continuous dosing of 1% of ethylene (blue curve), which is hydrogenated to ethane (green curve) under methanol (black curve) synthesis conditions, coupled with HPPEs with NH 3 . b Comparison of the continuous dosing of 0.05% NH 3 with the continuous dosing of 0.2% NO. The black bars describe the initial methanol mole fraction in pure syngas ( y MeOH, initial ) and in the presence of the corresponding impurity ( y MeOH, poisoned ). The red bars describe the dosed mole fraction of NH 3 ( y NH3, dosed ) and mole fraction in the product gas stream ( y NH3, effluent ). The blue bar (y NO, dosed ) stands for the dosed mole fraction of NO. X NH3 describes the corresponding degree of NH 3 conversion to the three methylamines: monomethylamine (orange bar), dimethylamine (grey bar) and trimethylamine (violet bar). c Syngas switching experiments from CO/CO 2 /H 2 to CO/H 2 and back to CO/CO 2 /H 2 at 210 °C and 60 bar coupled with HPPEs with NH 3 . Here, the resulting methanol (black curve) and NH 3 (green curve) mole fractions in the product gas stream are shown. The images visualize the oxidative effect of CO 2 in the syngas mixture and the corresponding interaction of NH 3 with the catalyst surface. Orange area = Cu 0 sites, blue area = Zn δ+ /ZnO sites, grey area = Zn 0 sites. Full size image Probing the presence of two different active sites From the first HPPEs, it can be seen that different types of N compounds interact with the active sites of the Cu/ZnO/Al 2 O 3 catalyst resulting in the observed decrease of methanol formation. Therefore, our work was focused on the identification of the nature of these active sites and on answering the question as to whether other surface sites play an important role. For these investigations, only the probe molecules NH 3 as reacting N compound (Fig. 2 ) and TMA as blocking N compound (Supplementary Fig. 12 ) were considered. The freshly reduced Cu/ZnO/Al 2 O 3 catalyst has various types of Lewis and Brønsted acid sites with different acid strengths. Actually, the Cu/ZnO/Al 2 O 3 catalyst developed for industrial reactors is a multi-site system. According to its composition, three different types of adsorption sites can be present [13] , [29] , [30] : the Cu–Zn interface, unpromoted metallic Cu 0 sites, and sites exposed by ZnO. In addition, every type of exposed surface is non-uniform due to the presence of vacancies, steps and kinks [13] . In general, the Cu:Zn ratio as well as the synthesis route is chosen in such a way that an intimate contact between Cu and ZnO is achieved to maximize the number of Cu–Zn interface sites. A significant influence of pure ZnO sites under the conditions of the low-temperature methanol synthesis can be neglected [31] , and the absence of acidic OH groups on the structural promoter Al 2 O 3 is also excluded due to the absence of acid-catalysed products such as dimethyl ether (Supplementary Note 3 ) [4] . For Al 2 O 3 , it is generally accepted that it acts as physical spacer to enhance the lifetime as well as the surface area of the Cu/ZnO catalyst maintaining economical methanol production rates over several years [4] . No evidence can be found in literature that Al 2 O 3 is involved in the reaction mechanism of methanol formation or in the formation of the active sites [32] , [33] . The hydrogenation of ethylene and NO was analysed in detail (Fig. 2a, b ) to identify the presence of different Cu sites, which has already been claimed in several publications [13] , [17] , [29] , [30] . 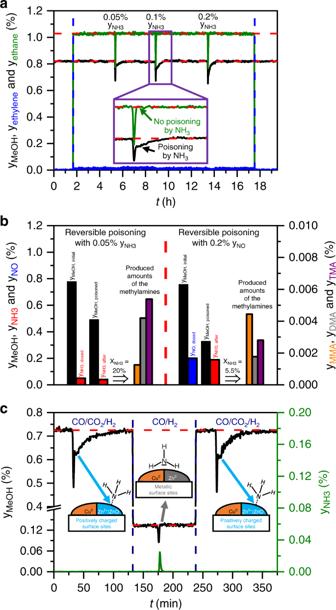Fig. 2: Continuous dosing experiments coupled with HPPEs. aContinuous dosing of 1% of ethylene (blue curve), which is hydrogenated to ethane (green curve) under methanol (black curve) synthesis conditions, coupled with HPPEs with NH3.bComparison of the continuous dosing of 0.05% NH3with the continuous dosing of 0.2% NO. The black bars describe the initial methanol mole fraction in pure syngas (yMeOH, initial) and in the presence of the corresponding impurity (yMeOH, poisoned). The red bars describe the dosed mole fraction of NH3(yNH3, dosed) and mole fraction in the product gas stream (yNH3, effluent). The blue bar (yNO, dosed) stands for the dosed mole fraction of NO.XNH3describes the corresponding degree of NH3conversion to the three methylamines: monomethylamine (orange bar), dimethylamine (grey bar) and trimethylamine (violet bar).cSyngas switching experiments from CO/CO2/H2to CO/H2and back to CO/CO2/H2at 210 °C and 60 bar coupled with HPPEs with NH3. Here, the resulting methanol (black curve) and NH3(green curve) mole fractions in the product gas stream are shown. The images visualize the oxidative effect of CO2in the syngas mixture and the corresponding interaction of NH3with the catalyst surface. Orange area = Cu0sites, blue area = Znδ+/ZnO sites, grey area = Zn0sites. Figure 2a shows that the continuous dosing of ethylene into the syngas stream leads to its nearly complete hydrogenation to ethane without influencing the rate of methanol formation. Thus, the two reactions are catalysed by two different active sites. Obviously, unpromoted metallic surfaces like Cu 0 are highly suitable for the hydrogenation of unsaturated hydrocarbons. It is known from literature that Cu 0 can act as adsorption site for ethylene [34] , and Cu-based catalysts are also applied in other hydrogenation reactions such as the hydrogenation of esters [35] . Furthermore, the high hydrogen content in the syngas is sufficient to ensure that ethylene hydrogenation can proceed without disturbing the formation of methanol on the Cu–Zn interface sites. Adding 0.05, 0.1 and 0.2% of NH 3 as pulses leads to the expected reversible poisoning of methanol formation, but not to a lowering of the produced amount of ethane neglecting the temporary dilution. The same result is obtained by comparing the continuous dosing of NH 3 with the continuous dosing of NO over the Cu/ZnO/Al 2 O 3 catalyst (Fig. 2b ). NO is completely hydrogenated to NH 3 and H 2 O, and the produced amount of NH 3 further reacts to methylamines (Supplementary Fig. 11 ). Figure 2b illustrates that a four times higher content of NO and so of the resulting NH 3 after hydrogenation compared with the added amount of 0.05% NH 3 leads to a degree of NH 3 conversion ( X NH3 ), which is nearly four times lower: 5.5% compared with 20%. This observation implies that NO is not hydrogenated on the same site where NH 3 reacts, that is, the NO hydrogenation sites are presumably metallic Cu 0 as for ethylene. Thus, the observed deactivation of methanol formation by adding NO originates from the re-adsorption of the hydrogenation products NH 3 and H 2 O, which is favoured under the applied high-pressure conditions according to the following consecutive reaction sequence [36] 
    NO→^ + H_2NH_3→^ + CH_3OHmethyl amines. (2) As a result, it seems that NH 3 does not prefer unpromoted metallic Cu 0 as adsorption site, which was also the outcome of NH 3 adsorption studies on Cu 0 single crystals [37] , [38] . To confirm this hypothesis, the syngas mixture was switched from CO/CO 2 /H 2 to CO/H 2 and back to the CO 2 -containing feed at constant reaction temperature and pressure, which is shown in Fig. 2c . The absence of CO 2 in the syngas mixture results in a strongly reducing atmosphere, which induces the formation of metallic surfaces on the Cu/ZnO/Al 2 O 3 catalyst. Increasing reaction temperatures and longer reaction times are known to result in brass formation [16] . Here, the lower production rates for methanol originate from a changed mechanism of methanol formation from the formate pathway to the formyl pathway, which is kinetically not preferred on Zn-promoted Cu 0 surfaces [17] . The adsorbates of the formyl mechanism such as CO ads and HCO ads bind through their C atoms to the catalyst surface, and no oxidising effect is induced due to the absence of CO 2 and H 2 O in contrast to the formate pathway. Therefore, the combination of this experiment with HPPEs shows no reversible poisoning and no conversion of NH 3 in the CO/H 2 mixture. Thus, the composition of the syngas mixture controls the oxidation state of the catalyst surface, which can be changed reversibly under low-temperature conditions as confirmed in many studies [11] , [16] , [24] . In summary, all experiments shown in Fig. 2 indicate that metallic Cu 0 or Cu 0 –Zn 0 sites are not the adsorption sites for NH 3 , implying that the observed reversible NH 3 poisoning in the presence of CO 2 must selectively proceed on positively charged Cu 0 –Zn δ+ interface sites due to the oxidising effect of the oxygen-containing adsorbates. The role of CO 2 It was already shown that adsorbates like formate or other oxygen-containing species originating from CO 2 play not only a crucial role in the methylation of amines, but also in the partial oxidation of Zn species in contact with metallic Cu 0 sites [12] , [13] . This type of oxidation is favoured for Zn due to its higher oxophilicity compared with Cu [13] , [17] . Providing evidence for this hypothesis requires that the corresponding investigations must be performed under high-pressure methanol synthesis conditions to generate the necessary adsorbates on the surface. For methanol synthesis over Cu/ZnO/Al 2 O 3 , the high-pressure pulse method combined with selective poisons as probe molecules enables us to analyse the oxidation effect under working conditions. For the investigation of the adsorbate-induced surface oxidation, the CO 2 content in the feed gas was increased from 0 (CO hydrogenation) to 100% (CO 2 hydrogenation) to generate different coverage degrees of the reaction intermediates, and for every gas mixture the normalized Δ n MeOH values (Supplementary Note 2 ) were determined by pulsing NH 3 and TMA (Fig. 3 ). Fig. 3: Influence of CO 2 on the methanol productivity and on the oxidation state of the catalyst surface. 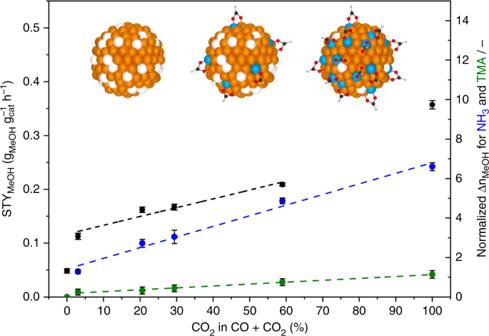Fig. 3: Influence of CO2on the methanol productivity and on the oxidation state of the catalyst surface. Correlation of the methanol productivity (black points and line) and of the normalized ΔnMeOHvalues (Supplementary Note2) of NH3(blue points and line) and TMA (green points and line) as a function of the CO2content in the syngas from pure CO hydrogenation (0%) to pure CO2hydrogenation (100%). Illustrations: Metallic Cu0particles (orange balls), metallic Zn0species (white balls), positively charged Zn species (blue balls) and formate as adsorbates. The error bars were determined by measuring every point five times. Correlation of the methanol productivity (black points and line) and of the normalized Δ n MeOH values (Supplementary Note 2 ) of NH 3 (blue points and line) and TMA (green points and line) as a function of the CO 2 content in the syngas from pure CO hydrogenation (0%) to pure CO 2 hydrogenation (100%). Illustrations: Metallic Cu 0 particles (orange balls), metallic Zn 0 species (white balls), positively charged Zn species (blue balls) and formate as adsorbates. The error bars were determined by measuring every point five times. Full size image Adding small amounts of CO 2 in the syngas feed results in a strong increase of the methanol production rate, which further increases with rising CO 2 content, because CO 2 is much faster hydrogenated to methanol than CO [17] . In general, it is accepted that the highest production rate is achieved at low CO 2 mole fractions around 2–4% [4] . This statement is only valid for high degrees of syngas conversion and high methanol and H 2 O mole fractions (Supplementary Fig. 13 ). In the differential kinetic regime, product inhibition effects by H 2 O are not significant enough to lower the rate of methanol formation strongly [17] , [36] . In addition to the increasing production rate of methanol, Fig. 3 illustrates that the observed poisoning strengths of NH 3 and TMA increase linearly as a function of the CO 2 content in the syngas mixture. Therefore, higher CO 2 mole fractions lead to increasing coverages of the resulting oxygen-containing adsorbates exemplary shown as formate, and these adsorbates create more Cu 0 –Zn δ+ interface sites. In this way, the adsorption capacity of TMA is enhanced, and more NH 3 molecules can be adsorbed and further converted. On the basis of the presented results and of different literature reports, we assume that the initial reduction of the catalyst surface induces the migration of metallic Zn species onto the metallic Cu 0 particles forming the Cu 0 –Zn 0 surface alloy [11] . This state of the surface seems to be stable under the conditions of CO hydrogenation, but not in the presence of CO 2 , which leads to the oxidation of the metallic Zn species forming Zn δ+ species on the Cu 0 surface [13] . It cannot be clarified if all Zn sites in contact with Cu 0 are oxidized in the CO 2 /H 2 gas mixture, but the majority of the sites should have a positively charged nature. The models of the active site of the Cu/ZnO/Al 2 O 3 catalyst of the Nakamura and Schlögl groups are rather similar proposing a Cu 0 –Zn 0 surface alloy [11] and Cu steps with Zn alloyed into it [13] , respectively. Behrens et al. [13] assumed the partial oxidation of the metallic Zn species, which cannot be neglected under industrially relevant coverage degrees. In contrast, the assumptions of the Nakamura and Chorkendorff groups [11] , [12] , [19] are mainly based on results obtained under atmospheric pressure or ultra-high vacuum, which result in low degrees of conversion and coverages. Thus, the fraction of oxidized Zn sites compared to the metallic ones is small, and the oxidation effect is hardly observable. For example, most characterization methods like our pulse experiments at 1 bar (Supplementary Fig. 9d ) provide an averaged result over the whole Cu surface area, which is mainly metallic. However, the Cu 0 –Zn 0 surface alloy model [11] provides a highly suitable description of the catalyst surface after reduction and presumably for methanol synthesis from CO. We analysed the rate of methanol formation reaction mainly from CO/CO 2 -containing syngas mixtures over an industrial Cu/ZnO/Al 2 O 3 catalyst, which can be reversibly deactivated by NH 3 , which initializes the consecutive methylation reactions. The step-by-step methylation with presumably oxygen-containing intermediates like formate seems to be the major factor determining the inhibition strength of the amines, because NH 3 is the strongest inhibitor. Both reactions selectively take place on the positively charged Zn species, which are formed by the diffusion of ZnO x species onto the metallic Cu 0 particles creating additional interface sites. The unpromoted Cu 0 sites act as hydrogenation sites for ethylene as well as NO, and sites exposed by ZnO nanoparticles are not active under the low-temperature conditions. For the hydrogenation products of NO, the re-adsorption of NH 3 and H 2 O is favoured under the high-pressure conditions. In addition, we showed that the CO 2 content in the syngas is essential to achieve the optimum oxidation state of the interface sites, which are less active and more metallic in the absence of CO 2 . The resulting adsorbate-induced oxidation of surface sites by formate and the importance of Lewis acids on metallic Cu 0 for the formation of methanol were also observed in recent studies [39] , [40] . Actually, the statement that CO 2 is important for the oxidation state of the surface goes back to Klier et al. [41] , who assumed erroneously that Cu + is the active site. 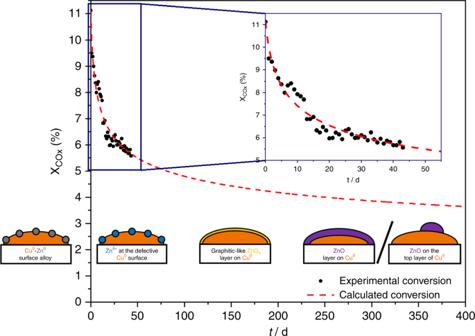Fig. 4: Long-term methanol synthesis over the industrial Cu/ZnO/Al2O3catalyst at 210 °C and 60 bar. Recorded degrees of conversion (black points) under differential controlled conditions. The dashed red curve describes the intra- and extrapolation of the experimental data, which was calculated with the MATLAB®software according to the studies of Fichtl et al.18. Illustrations from right to left: Cu0–Zn0surface alloy according to Nakamura et al.11. Znδ+species at the defective Cu0surface according to Behrens et al.13, graphitic-like ZnOxlayer on Cu0according to Lunkenbein et al.14. ZnO layer on Cu0according to Lunkenbein et al.23as well as Fichtl et al.18and ZnO on the top layer of Cu0according to Kattel et al.15. Figure 4 illustrates that all newer models can be applied to describe the structural evolution of the Cu/ZnO/Al 2 O 3 catalyst as a function of TOS. Fig. 4: Long-term methanol synthesis over the industrial Cu/ZnO/Al 2 O 3 catalyst at 210 °C and 60 bar. Recorded degrees of conversion (black points) under differential controlled conditions. The dashed red curve describes the intra- and extrapolation of the experimental data, which was calculated with the MATLAB ® software according to the studies of Fichtl et al. [18] . Illustrations from right to left: Cu 0 –Zn 0 surface alloy according to Nakamura et al. [11] . Zn δ+ species at the defective Cu 0 surface according to Behrens et al. [13] , graphitic-like ZnO x layer on Cu 0 according to Lunkenbein et al. [14] . ZnO layer on Cu 0 according to Lunkenbein et al. [23] as well as Fichtl et al. [18] and ZnO on the top layer of Cu 0 according to Kattel et al. [15] . Full size image The strong loss of ~50% of the initial activity in the first weeks is inevitable for Cu-based catalysts developed for industrial reactors due to thermal sintering and restructuring [4] . Therefore, the Cu/ZnO/Al 2 O 3 catalyst is a dynamic system with a continuously changing structure, so that true steady state for a couple of days cannot be reached even under industrial timescales as illustrated by the extrapolated curve. We propose the following structural changes as a function of TOS from left to right in Fig. 4 : At the beginning, highly reduced ZnO x species migrate onto the metallic Cu 0 nanoparticles during reduction forming a finely dispersed Cu 0 –Zn 0 alloy according to Nakamura et al. [11] . The change to a CO 2 -containing syngas mixture initializes the formation of different oxygen-containing adsorbates as well as the oxidation of the metallic Zn species to Zn δ+ species at the defective Cu 0 surface according to Behrens et al. [13] . The migration of further Zn species results in the formation first of a graphitic-like ZnO x layer on Cu 0 according to Lunkenbein et al. [14] and then a more crystalline and stable thick ZnO layer or particles according to Kattel et al. [15] . The formation of thick ZnO layers due to segregation from the metallic Cu 0 phase were observed in recent long-term studies [18] , [23] clarifying that the SMSI process is thermodynamically preferred, but kinetically slow. Under industrially relevant conditions our results clearly confirm the presence of highly active Cu 0 –Zn δ+ interface sites embedded in the structurally constantly changing matrix provided by the Cu/ZnO/Al 2 O 3 catalyst Thus, by applying our developed high-pressure pulse method, we were able to identify the nature of these interface sites, which has not been possible by other characterization methods lacking the combination of surface sensitivity and industrially relevant reaction conditions. Activation and aging of the Cu/ZnO/Al 2 O 3 catalyst All measurements in this work were performed with the same industrial Cu/ZnO/Al 2 O 3 catalyst provided by Clariant Produkte (Deutschland) GmbH using a standard high-pressure flow set-up including mass flow controllers (MFC, Bronkhorst Deutschland Nord GmbH) for the adjustment of the necessary volume flows, shutdown (Swagelok Company) and multi-port (VICI Valco Instruments) valves, one tubular 1/4-inch stainless-steel reactor mounted in a 1-zone oven (HTM Reetz GmbH) and equipped with an internal thermocouple in order to achieve the desired reaction temperature in the catalyst bed, a back pressure regulator (BPR, Equilibar Precision Pressure Control) connected to a process pressure controller (PC, Bronkhorst Deutschland Nord GmbH) for the reaching of high-pressure conditions (up to 60 bar) in the reactor and a unique self-built HPPU. In addition, all stainless-steel tubes and parts, which were contaminated by the corrosive reversible poisons used in this work, were coated with SilcoNert 2000® provided by SilcoTek GmbH and heated up to 150 °C to minimize any kind of adsorption phenomena. For the quantification of the product gas streams, a combination of a FTIR spectrometer (Nicolet is50, Thermo Fisher Scientific) and a Micro GC device (Micro GC 490, Agilent) was used. The spectrometer contains a transmission gas cell in the sample holder with ZnSe windows, a pathlength of 150 mm and a cell volume of 7.5 ml. In addition, the spectrometer offers two different types of detectors for recording IR spectra: The thermal DTGS (deuterated triglycine sulfate) and the liquid nitrogen cooled MCT (mercury cadmium telluride) detectors. In the case of the Micro GC device, a pump, a micro-machined injector with an injection volume of 5 µl, a Molsieve 5A column and a micro-machined thermal conductivity detector were used for recording the chromatograms. The calibrations of both analytics were validated and the carbon balance (C-balance) of every kinetic experiment performed in this work was in the acceptable range of 100% ± 1%. C - balance = y_C,out/y_C,in = y_CO,out + y_CO2,out + y_MeOH,out/y_CO,in + y_CO2,in. (3) Here, the ratio between the mole fraction of all carbon-containing compounds (CO, CO 2 , CH 3 OH) in the product gas stream y c, out and the mole fraction of all carbon-containing compounds (CO, CO 2 ) in the feed y c, in yields the C-balance. For the reduction of the catalyst precursor, the temperature was increased to 175 °C with a heating rate of 1 °C min −1 using a gas flow rate of 500 Nml min −1 g cat −1 diluted H 2 (2% H 2 (99.999%) in N 2 (99.999%)) for 15 h. In a second step, the temperature was increased to 240 °C with 1 °C min −1 and held for 30 min. After the second increase of the temperature, the reduced catalyst was ready for methanol synthesis. To reach steady-state conditions in a relatively short period of time, the catalyst was aged before performing the kinetic experiments. The reaction temperature was increased to 250 °C at 60 bar to establish equilibrium-controlled conditions ensuring a reproducible deactivation by exposing the whole catalyst bed to the same gas composition at high degrees of conversion according to the study by Fichtl et al. [18] . As standard syngas mixture, the following composition was used: 13.5% CO (99.997%), 3.5% CO 2 (99.998%), 73.5% H 2 (99.999%) and 9.5% N 2 (99.999%). All measurements in this study were performed in the differential regime with the necessary syngas flow rate. High-pressure pulse experiment (HPPE) For the HPPE, a self-built HPPU was developed to inject probe molecules as pulses under high-pressure conditions, which is schematically shown in Fig. 5 . Fig. 5: Scheme of the high-pressure pulse unit integrated in the flow set-up. PI is defined as pressure sensor in the corresponding line. The area in blue describes the flow direction of the syngas mixture, the red area of the injected impurities and the orange area of the reference gas (Ar) for pressure regulation. Full size image The HPPU consists of one 6 port, 2 position valve equipped with a 1 ml sample loop and two identical back pressure regulators (BPR1 and BPR2) coupled with one process PC. BPR2 is integrated in the reactor line between the reactor outlet and the analytics and BPR1 in the pulse line between the sample loop and the exhaust. The method for the injection of a pulse over the catalyst bed in the reactor under high-pressure conditions is as follows: The BPRs consist of two parts, which are separated from each other by a Kapton ® membrane. The upper parts are connected with PC and the other parts with the incoming gas flow from the reactor or the sample loop on the inlet sites and on the outlet sites with the analytics or exhaust. The task of the PC is to reach the same pressure level in both back pressure regulators. It consists of two valves and a pressure sensor PI. For the setting of pressure values up to 60 bar, 65 bar of Ar (99.999%) must be connected on the inlet valve. When a pressure value is set in the program of the PC, the inlet as well as outlet valve is opened and closed until the pressure sensor measures the given value. Consequently, the pressure in both upper parts of BPR1 and BPR2 increases and so the membranes are pressed down. 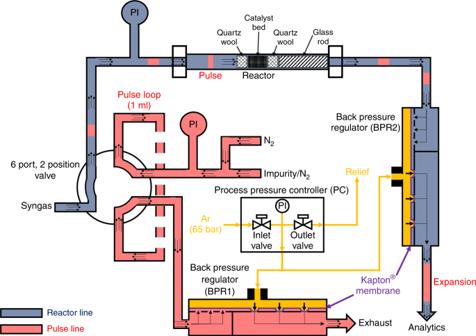Fig. 5: Scheme of the high-pressure pulse unit integrated in the flow set-up. PI is defined as pressure sensor in the corresponding line. The area in blue describes the flow direction of the syngas mixture, the red area of the injected impurities and the orange area of the reference gas (Ar) for pressure regulation. At this moment, the gas flows are stopped and the pressure in the reactor line and pulse line builds up until the same pressure level is reached like in the upper parts. Then, the membranes are lifted up to the starting positions and the gas mixtures can flow again. If both pressure sensors PI in the reactor and pulse line show the same pressure value, then the valve can be switched to inject the first pulse into the syngas stream. The results of the validation are shown in Fig. 6 . Here, 200 mg of α-Al 2 O 3 (sieve fraction: 250–355 µm, Südchemie GmbH) were placed in the isothermal zone of the reactor and fixed between two plugs of quartz wool to simulate an inert catalyst bed. One glass rod was placed after the bed to lower the dead volume. Then, 0.3% CH 4 (99.995%) in N 2 (99.999%) as IR-active, but inert gas was injected as pulses into a 50 Nml min −1 N 2 (99.999%) flow passing through the α-Al 2 O 3 bed at 5, 10, 20, 30, 40, 50 and 60 bar. The retention time τ and the pulse area A pulse of the recorded pulses (Fig. 6a ) were determined and correlated with the set pressures (Fig. 6b ). Fig. 6: Validation of the self-built high-pressure pulse unit with inert CH 4 pulses over α-Al 2 O 3 . a Recorded methane pulses (green curves) injected over α-Al 2 O 3 as inert bed at different pressures from 5 to 60 bar. τ is defined as the retention time of the CH 4 pulses. b Correlation of the determined retention times τ (red points and line) and pulse areas A pulse (blue points and line) against the set pressure levels. The error bars were determined by measuring every point 5 times. Full size image The dashed red line in Fig. 6a represents the injection point of the pulses at time 0. Increasing the pressure leads to longer τ and increasing A pulse . In this case, only the blue curve ( A pulse ) in Fig. 6b goes through the origin and not the red curve ( τ ). The reason for this is the constant operation of the analytics under atmospheric pressure and so the expansion of the pulses after the BPR2 (Fig. 5 ). In general, the volume flow \(\dot V\) of gaseous compounds is reduced by increasing the pressure level p according to the ideal gas law (Eq. ( 4 )), since the molar flow \(\dot n\) (due to a constant mass flow provided by the used MFC at every pressure level), the gas constant R and the temperature T (due to small changes in the pressure level) can be seen as constant: 
    p = ṅ· R · T/V̇ = const. ·1/V̇
 (4) 
    τ = V/V̇ = const. · p
 (5) In contrast, the resulting retention time or residence time τ , which is defined as reactor volume V divided by the volume flow \(\dot V\) of the pulses is proportional to the applied pressure. The corresponding value for the constant in Eq. ( 5 ) is equal to the slope m of the lines in Fig. 6b . The linear behaviour of both functions (Fig. 6b ), the absence of steps in the recorded pulses and the acceptable tailing at higher pressures (Fig. 6a ) demonstrate a successful validation of the HPPU. Consequently, significant pressure drops and backmixing of the probe molecules can be excluded. In addition, the small error bars (every measurement was repeated five times) in Fig. 6b underline the reproducibility of the pulse method. For a typical HPPE, 100 mg of the industrial Cu/ZnO/Al 2 O 3 catalyst (sieve fraction 250–355 µm) were placed in the tubular reactor. In the first step, the initial methanol mole fraction in the standard syngas mixture at 210 °C and 60 bar was recorded under differential controlled conditions. Then, the different N compounds were injected as pulses from the corresponding gas cylinder: 0.5% NH 3 (99.999%) in N 2 (99.999%), 0.2% NO (99.5%) in N 2 (99.999%), 0.2% monomethylamine (MMA, 99.5%) in N 2 (99.999%), 0.2% dimethylamine (DMA, 99.5%) in N 2 (99.999%), 0.2% trimethylamine (TMA, 99.5%) in N 2 (99.999%). The mole fraction in the sample loop was set at 0, 0.01, 0.025, 0.05, 0.075, 0.1 and 0.2%. The measurement with 0% corresponds to a pulse with pure inert gas N 2 (99.999%). In the case of NH 3 , additional HPPEs were performed with 0.4 and 0.5%. In addition, 0.05, 0.1 and 0.2% NH 3 were injected at 230 and 250 °C at constant 60 bar as well as at 1, 10, 30 and 60 bar at constant 210 °C. Co-feeding of NH 3 , NO, MMA, DMA and TMA The continuous dosing experiments with various N compounds were performed over 200 mg (sieve fraction 250–355 µm) of the industrial methanol catalyst. For the dosing of 0.05% NH 3 (from 0.5% NH 3 (99.999%) in N 2 (99.999%)) and 0.2% NO (from 2% NO (99.5%) in N 2 (99.999%)), the reaction temperature and pressure were set at 210 °C and 60 bar. In the case of dosing of 0.051% NH 3 , 0.0153% MMA (from 0.2% MMA (99.5%) in N 2 (99.999%)), 0.0170% DMA (from 0.2% DMA (99.5%) in N 2 (99.999%)) and 0.0157% TMA (from 0.2% TMA (99.5%) in N 2 (99.999%)), the reaction temperature was increased to 250 °C. After achieving a constant initial methanol mole fraction applying the standard syngas mixture, the corresponding N compound was continuous dosed over the catalyst bed for a defined period of time by replacing the internal standard N 2 in the standard syngas mixture. At the end, the gas stream of the N compounds was switched off to measure the methanol activity in pure syngas. Co-feeding of ethylene coupled with HPPE with NH 3 /TMA The combination of methanol synthesis in the presence of ethylene coupled with HPPEs with NH 3 and TMA were performed with 100 mg of the industrial Cu/ZnO/Al 2 O 3 catalyst (sieve fraction 250–355 µm) mounted in the tubular reactor. In the first step, the initial methanol mole fraction was determined with the standard syngas mixture at 210 °C and 60 bar. Then, 1% of the internal standard N 2 was replaced by ethylene (from 20% ethylene (99.995%) in N 2 (99.999%)) and after a defined period of time, the feed was switched back to the standard syngas mixture. During the adding of ethylene, 0.05%, 0.1% and 0.2% of NH 3 (from 0.5% NH 3 (99.999%) in N 2 (99.999%)) and TMA (from 0.2% TMA (99.5%) in N 2 (99.999%)) were injected as pulses. Syngas switching experiments coupled with HPPE with NH 3 /TMA The combination of syngas switching experiments under methanol synthesis conditions with HPPEs with NH 3 and TMA were carried out over 100 mg of the industrial Cu/ZnO/Al 2 O 3 catalyst (sieve fraction 250–355 µm). Here, the syngas feed was changed from the standard mixture containing CO/CO 2 to 17% CO (99.997%), 73.5% H 2 (99.999%), 9.5% N 2 (99.999%) and back to the standard mixture. At each instant, methanol was produced at 210 °C and 60 bar. In addition, pulses containing 0.2% of NH 3 (from 0.5% NH 3 (99.999%) in N 2 (99.999%)) and TMA (from 0.2% TMA (99.5%) in N 2 (99.999%)) were injected into the different feed gas compositions. CO/CO 2 variation experiment coupled with HPPE with NH 3 /TMA The combination of CO/CO 2 variation experiments under methanol synthesis conditions with HPPEs with NH 3 and TMA were performed with 100 mg of the Cu/ZnO/Al 2 O 3 catalyst (sieve fraction 250–355 µm) in the tubular reactor. The reaction temperature and pressure were constant at 210 °C and 60 bar and the CO 2 content in the syngas feed was changed from 0 to 17% (0, 0.5, 3.5, 5, 10, 17%) by substituting or adding CO to maintain the carbon mole fraction at constant 17% (CO + CO 2 ). For every new syngas mixture, the methanol productivity was recorded and 0.2% NH 3 (from 0.5% NH 3 (99.999%) in N 2 (99.999%)) as well as TMA (from 0.2% TMA (99.5%) in N 2 (99.999%)) were injected as pulses. Every measurement was repeated five times to determine the corresponding error bars. Long-term measurement The procedure of the long-term measurement was adapted from Fichtl et al. [18] . and is shown in Fig. 7 . Fig. 7: Experimental protocol of the long-term measurement adapted from the studies by Fichtl et al. [18] . 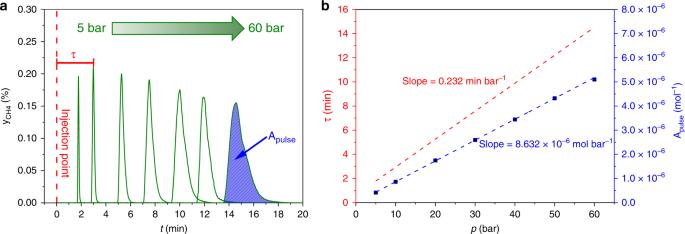Fig. 6: Validation of the self-built high-pressure pulse unit with inert CH4pulses over α-Al2O3. aRecorded methane pulses (green curves) injected over α-Al2O3as inert bed at different pressures from 5 to 60 bar.τis defined as the retention time of the CH4pulses.bCorrelation of the determined retention timesτ(red points and line) and pulse areasApulse(blue points and line) against the set pressure levels. The error bars were determined by measuring every point 5 times. 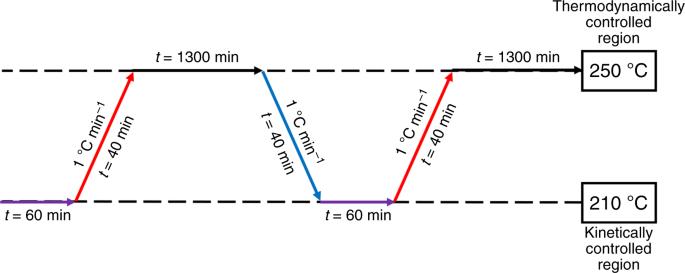Fig. 7: Experimental protocol of the long-term measurement adapted from the studies by Fichtl et al.18. The violet arrow describes the period of time to record the kinetic data point, the red arrow describes the heating rate, the black arrow describes the aging of the catalyst bed under equilibrium conditions and the blue arrow describes the cooling rate. The violet arrow describes the period of time to record the kinetic data point, the red arrow describes the heating rate, the black arrow describes the aging of the catalyst bed under equilibrium conditions and the blue arrow describes the cooling rate. Full size image Three hundred milligrams of the industrial methanol synthesis catalyst (sieve fraction 250–355 µm) were mixed with 1800 mg purified α-Al 2 O 3 (sieve fraction 510–750 µm) and placed in the tubular reactor. The high dilution should prevent the formation of hot spots, so that a homogeneous temperature profile over the entire catalyst bed was obtained. After the standard activation procedure, the gas stream was changed to the standard syngas mixture and the reaction pressure was increased up to 60 bar. The initial activity test was performed at 210 °C for 60 min under kinetically controlled conditions. Then, the catalyst was heated to the aging temperature of 250 °C and the volume flow was reduced to reach the equilibrium conversion. The equilibrium condition was held for 90% of a day. The decrease of the reaction temperature to 210 °C and the increase of the flow rate allowed to measure the next kinetically controlled rate of methanol formation. The continuous change between the two conditions was carried out until a total TOS of 6 weeks was reached. Besides, the recorded experimental curve was interpolated by using the following empirical power-law model (PLM): 
    da_rel/dt = - k_d · a_rel( t )^m,
 (6) 
    a_rel = X_COx(TOS)/X_COx(TOS = 0),
 (7) a rel is defined as the relative activity, the ratio between the time-dependent CO x (CO + CO 2 ) conversion ( X CO x ( TOS ) ) and the CO x conversion of the initial activity ( X CO x (TOS = 0)). k d is the deactivation rate constant and m is an empirical factor or the reaction order. For the calculation of the theoretical curve, the MATLAB ® software was used and the procedure was adapted from the work of Fichtl et al. [18] .